A dynamic supramolecular polymer with stimuli-responsive handedness forin situprobing of enzymatic ATP hydrolysis Design of artificial systems, which can respond to fluctuations in concentration of adenosine phosphates (APs), can be useful in understanding various biological processes. Helical assemblies of chromophores, which dynamically respond to such changes, can provide real-time chiroptical readout of various chemical transformations. Towards this concept, here we present a supramolecular helix of achiral chromophores, which shows chiral APs responsive tunable handedness along with dynamically switchable helicity. This system, composing of naphthalenediimides with phosphate recognition unit, shows opposite handedness on binding with ATP compared with ADP or AMP, which is comprehensively analysed with molecular dynamic simulations. Such differential signalling along with stimuli-dependent fast stereomutations have been capitalized to probe the reaction kinetics of enzymatic ATP hydrolysis. Detailed chiroptical analyses provide mechanistic insights into the enzymatic hydrolysis and various intermediate steps. Thus, a unique dynamic helical assembly to monitor the real-time reaction processes via its stimuli-responsive chiroptical signalling is conceptualized. Helically organized polymeric [1] , [2] , [3] and supramolecular [4] , [5] , [6] , [7] assemblies have been the subject of considerable interest as biomimetic systems to understand and appreciate asymmetric preferences like homochirality in nature. Typical designs of helical assemblies consist of optically active monomers, which bias the handedness during the (supramolecular) polymerization process [8] , [9] , [10] , [11] , [12] , [13] , [14] , [15] , [16] , [17] , [18] , [19] . In this respect, helicity induction in racemic or achiral assemblies constructed from achiral monomers through non-covalent interactions with the chiral guest molecules is an alternative, synthetic strategy [20] , [21] , [22] , [23] , [24] , [25] , [26] . This host–guest design for helical motifs not only provides new opportunities to investigate mechanistic details of supramolecular chirality, but also offers practical chirotechnological applications. For example, this design has been used for the asymmetric synthesis of metastable homochiral systems (chiral memory) from kinetically stable assemblies, by the post-synthetic removal of chiral guest molecules (auxiliaries) [27] , [28] , [29] , [30] , [31] . In particular, this approach has helped to understand the mechanistic pathways of racemization and various off-nucleation processes of supramolecular polymers [32] , [33] . On the other hand, dynamic helical assemblies, with stimuli-responsive chiroptical and conformational responses have been used as enantioselective sensors and actuators [34] , [35] , [36] , [37] , [38] . Another advantage, which can be envisaged of dynamic helical assembly, is their real-time chiroptical readout in response to various processes and stimuli influencing the assembly [39] . Adenosine phosphates (APs) are key biologically relevant chiral molecules, which define the energy economy of most living systems [40] . They exist in various forms like ATP, ADP, AMP and their interconversion phenomena is directly related to various processes occurring in the living cell. To probe the interconversion of AP, that is, AMP or ADP or ATP, specific signalling is required and hence dynamic helical systems, which can differentially respond to these chiral phosphates, provide a viable alternative. In this work, we present a supramolecular helical assembly that responds to various AP with a differential chiroptical signalling, which is utilized for probing an enzymatic reaction in real time. This system comprises of self-assembled naphthalenediimide (NDI) chromophores, end functionalized with zinc coordinated dipicolylethylenediamine receptor motifs (NDPA) [41] , which show induction of opposite handedness on binding to AMP or ADP when compared with ATP ( Fig. 1 ) [42] . Very fast response to change of binding guests as well as lack of chiral amplification makes the chosen assembly most suited to study the real-time in situ conversion kinetics of AP from one form to another, which was further proven conceptually by the enzymatic hydrolysis of ATP. The utilization of supramolecular handedness as a probe, not only to monitor enzymatic ATP decay but also to follow its course of stepwise conversion to ADP, AMP and finally to phosphates, is unprecedented and provides useful insight into the hydrolytic pathway. In addition, this strategy also provides a unique way to control the stereomutation rates of helical assemblies by changing the concentrations of external stimuli. 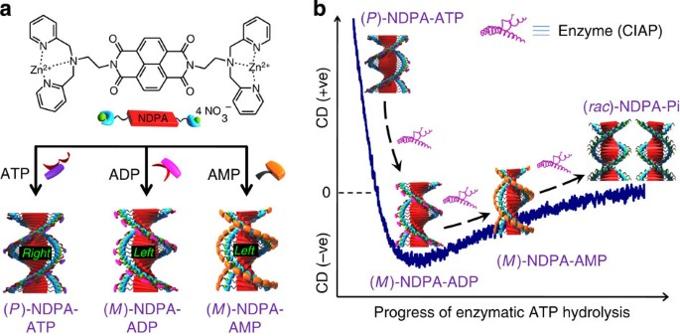Figure 1: Enzyme-responsive helical handedness of NDPA-ATP/ADP/AMP/Pi supramolecular polymer. (a) Molecular structure of NDPA along with the pictorial representation of adenosine phosphates (AP) induced helical supramolecular organization. (b) Schematic illustration of the dynamic helix reversals upon enzyme (CIAP) action on the NDPA-bound ATP molecules and their respective real-time chiroptical readout. Figure 1: Enzyme-responsive helical handedness of NDPA-ATP/ADP/AMP/Pi supramolecular polymer. ( a ) Molecular structure of NDPA along with the pictorial representation of adenosine phosphates (AP) induced helical supramolecular organization. ( b ) Schematic illustration of the dynamic helix reversals upon enzyme (CIAP) action on the NDPA-bound ATP molecules and their respective real-time chiroptical readout. Full size image Differential chiroptical response Very recently, we described the one-dimensional supramolecular polymerization of NDPA in water by the molecular recognition of various AP [42] . The absorption spectrum of NDPA shows sharp bands ( λ max =381 and 361 nm), characteristic of NDI chromophores devoid of intermolecular interactions and are indicative of monomeric nature of these chromophores. Binding of anionic AP to cationic NDPA resulted in stacking of NDI chromophores via synergistic hydrophobic and π–π interactions, characterized by the broadening of absorption band, along with the intensity reversal of vibronic bands ( Supplementary Fig. 1 ). Chiroptical probing of these co-assembled stacks with circular dichroism (CD) spectroscopy showed strong bisignated Cotton effects and are indicative of a helical bias in the supramolecular organization of achiral NDIs induced by homochiral AP. The mode of binding probed through CD Job plot and titrations showed that AMP, ADP and ATP bind through one, two and three point of attachment, respectively [42] . Also, comparative absorption spectra show that the interchromophoric interactions are strongest upon ATP binding followed by ADP and weakest by AMP, as evident from their change in intensity ratio ( I 0-0 / I 0-1 ) of two lower energy vibrational transitions ( Supplementary Fig. 1 ). Interestingly, AMP and ADP imparted M -helicity (left-handed) to the NDPA stacks, as evident from the negative bisignated CD signal, whereas ATP induced P -helicity (right-handed) with positive bisignated CD signal ( Fig. 2a ). 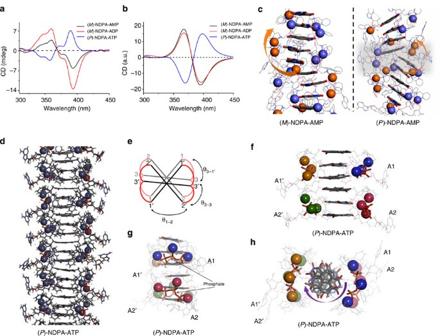Figure 2: AP-induced reverse helical assembly of NDPA. (a) Experimental CD spectra and (b) average trace of simulated CD spectra on several conformations extracted from MD runs of NDPA-AMP, NDPA-ADP and NDPA-ATP. Opposite bisignated Cotton effects with various AP indicates their reverse handedness. (c) Inner structure of(M)-NDPA-AMP and(P)-NDPA-AMP assemblies obtained at the end of MD. The shaded region highlights stacking defects inP-helix. (d–h) Inner structure of(P)-NDPA-ATP at the end of MD. (d) A portion of the assembly; (e) schematic representing top view of two stacked trimers, showing ATP-forming 1-3-2 motif in red and the angles between successive NDI along the stack (NDIs are numbered with 1, 2, 3 for bottom, middle and top molecules in a trimer, respectively. Similarly, 1′, 2′, 3′ is for the second trimer). (f) Front view, (g) side view and (h) top view of two trimers (A=adenine) of(P)-NDPA-ATP. Inc,f–h, the Zn atoms are depicted in balls, with different colours depending on which side of NDPA they are located, to show chirality of the assembly. NDPA are depicted in thick sticks and H-bonds in dashed light blue lines. Inc,h, the arrows guide the eye to show chirality (pointing towards the back of the view). Figure 2: AP-induced reverse helical assembly of NDPA. ( a ) Experimental CD spectra and ( b ) average trace of simulated CD spectra on several conformations extracted from MD runs of NDPA-AMP, NDPA-ADP and NDPA-ATP. Opposite bisignated Cotton effects with various AP indicates their reverse handedness. ( c ) Inner structure of (M) -NDPA-AMP and (P) -NDPA-AMP assemblies obtained at the end of MD. The shaded region highlights stacking defects in P -helix. ( d – h ) Inner structure of (P) -NDPA-ATP at the end of MD. ( d ) A portion of the assembly; ( e ) schematic representing top view of two stacked trimers, showing ATP-forming 1-3-2 motif in red and the angles between successive NDI along the stack (NDIs are numbered with 1, 2, 3 for bottom, middle and top molecules in a trimer, respectively. Similarly, 1′, 2′, 3′ is for the second trimer). ( f ) Front view, ( g ) side view and ( h ) top view of two trimers (A=adenine) of (P) -NDPA-ATP. In c , f – h , the Zn atoms are depicted in balls, with different colours depending on which side of NDPA they are located, to show chirality of the assembly. NDPA are depicted in thick sticks and H-bonds in dashed light blue lines. In c , h , the arrows guide the eye to show chirality (pointing towards the back of the view). Full size image Molecular dynamics simulation for differential helicity To understand the origin of opposite handedness in NDPA assembly on AMP or ADP binding when compared with ATP binding, detailed molecular mechanics (MM)/molecular dynamics (MD) simulations were performed ( Supplementary Figs 2–5 , Supplementary Notes 1 and 2 ). With AMP, the comparison of potential energy profiles on 20 ns MD runs shows that the M -helices, that is, (M) -NDPA-AMP, are 1.5–2.4 kcal per mole per molecule more stable than P -helices, (P) -NDPA-AMP ( Supplementary Table 1 , Supplementary Note 1 ). The main contribution of such energy differences between two helices originates from non-bonding (mostly van der Waals) interactions. A better global and local ordering exists in the left-handed helix over the right analogue, as suggested by a smaller average distance between successive NDPA (4.0 Å versus 4.4 Å), more π–π contacts per molecule, smaller deviations in average distances and rotational strengths between successive NDPA, and the presence of stacking defects in P -helix compared with M -helix ( Fig. 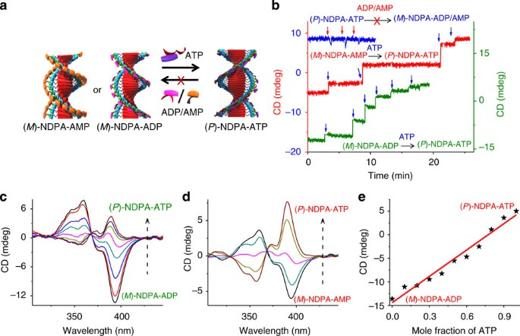Figure 3: Dynamic helix reversal and chiral amplification. (a) Pictorial representation of helicity reversal in NDPA assembly via competitive binding of multivalent AP. (b–d) Stepwise dynamic helix reversal experiments performed by sequential addition of ATP to(M)-NDPA-AMP and(M)-NDPA-ADP assemblies (5 × 10−5M NDPA in aqueous HEPES (2-[4-(2-hydroxyethyl)piperazin-1-yl]ethanesulfonic acid) with 1 equivalent of respective phosphates). (b) Green and red traces show the sharp jumps in CD signal intensity of(M)-NDPA-AMP and(M)-NDPA-ADP, respectively, monitored at 394 nm, upon sequential addition of ATP, represented by the blue arrows. These sharp rises in CD intensity are characteristic of fast helicity reversal and the formation of(P)-NDPA-ATP stacks, which is further evident from the corresponding CD spectral changes shown inc,d. Horizontal nature of these traces suggest that waiting time does not affect the intensity. Blue trace inbshows the CD intensity of(P)-NDPA-ATP upon sequential addition of AMP at time intervals as indicated by the red arrows. The retention of handedness suggests the inability of AMP to replace the pre-bound ATP molecules. (e) ‘Majority rules’ like experiment performed using a mixture of ADP and ATP. The linear fit (red line) of the CD intensity rules out any chiral amplification. 2c shaded region, Supplementary Table 3 ). This improvement of ordering is attributed to the orientation of the chiral ribose moieties, which is related to their chirality. In the M -helix, the ribose moieties are close to the NDPA cores, whereas in the P -helix, they are oriented at the periphery of the stack ( Fig. 2c ). With this proximity in the M -Helix, the hydroxyl groups of ribose moieties form hydrogen bonding with the oxygen atoms of NDPA. These interactions can take place between molecules n and n +2 or n +3, thus contributing to long-range ordering of the assembly. Up to two such hydrogen bonds per molecule occur in the M -helix, which is three times higher than in the P -helix ( Supplementary Table 2 ). The simulated CD spectrum of (M) -NDPA-AMP ( Fig. 2b, Supplementary Methods ) shows a negative bisignated signal with zero crossing around 380 nm, and positive and negative maxima at 367 and 395 nm, respectively, in good agreement with experimental spectra. With ADP, similar observations to AMP were made both in terms of energy and morphology. The M -helices are slightly more stable than P -helices (by 0.5 kcal per mol per molecule). The rotation angle between successive NDPA-ADP is around 58°±10°, similar to what is found for NDPA-AMP (57°±11°), that is, around 6.3 NDPA per turn for both systems ( Supplementary Fig. 6 ). The stacking distance of NDPA is slightly reduced from 4.0 to 3.8 Å, from AMP to ADP, likely due to the extra constraint imposed by ADP on adjacent molecules, which form dimers. The simulated CD spectrum for (M) -NDPA-ADP ( Fig. 2 ) shows a negative bisignated signal with zero crossing around 380 nm. This result is similar to the one obtained with AMP and in close agreement with the experimental CD signal. ATP offers far more binding possibilities, and hence more assemblies than AMP or ADP. However, two families of assemblies emerged from the simulations, depending on the binding motif: 1-2-3 or 1-3-2. This numbering refers to the stacking order and binding motif. The molecules are numbered along the stacking direction: X-Y-Z motif means that the NDPA molecules form trimers, where molecule X is linked to molecule Y, which is linked to molecule Z ( Fig. 2e for the 1-3-2 motif, Supplementary Fig. 7 , Supplementary Note 3 ). The most stable structures were obtained for assemblies with 1-3-2 binding motif ( Supplementary Figs 8 and 9 ). Although the NDI cores do form a helical assembly (six NDIs per turn), the Zn-triphosphate complexes form two columns on both sides of the central helix ( Fig. 2d–h ). As the pitch of NDI helix is similar with any AP (6 molecules with ATP, versus ~6.3 with AMP or ADP), as well as the average rotation angle between neighbouring molecules (60° versus 57–58°, respectively), the columnar arrangement of complexes is to be explained by symmetry. With AMP, the angle between the AP complexes is the same as the angle between the NDIs, and thus the complexes also form an helix. With NDPA-ATP, because each complex with ATP involves three NDIs, the angle between the complexes (trimers) is three times the angle between the NDIs, that is, about 180°. As a result, the assembly of AP complexes has a pitch of only two complexes, and thus appears columnar where the trimers are translational images from each other along the stacking direction. We then investigated in more detail a representative 1-3-2 right-handed assembly. Although the average angle between NDIs is of 60°, a more detailed analysis reveals that there are three population distributions: the angle between molecules 1 and 2, θ 1-2 is 81°±4°. Similarly, θ 2-3 is 44°±4° and θ 3-1′ =54°±4°, 1′ refering to a molecule belonging to a neigbouring trimer ( Fig. 2e–g ). The first two angles deviate from the angle found in the NDPA-AMP arrangement (~57°), because of the constraints imposed by ATP. The third one, however, measured between molecules belonging to adjacent trimers, that is, molecules more free to rotate with respect to each other, is not much affected. This result indicates weak steric hindrance between trimers, which are able to stack while conserving the natural angle between single NDPA molecules. The sum of the three angles is 179°, corresponding well to the symmetry condition necessary for having AP complexes forming columns instead of helices. Experimentally, for NDPA-ATP, P -helices are more stable than the M -helices, which is opposite to the situation with AMP and ADP. As the organization within the NDI stacks is rather similar in the three systems, the change of helicity has to be found in the AP complexes. Their organization is indeed very different in AMP or ADP systems when compared with ATP systems. With AMP and ADP in left-handed structures, the adenosine moieties are close enough to NDI cores to form H-bonds, principally via the hydroxyl groups. However, these interactions do not exist in the ATP systems as the adenosine moieties are pointing away ( Fig. 2d–f ). This is illustrated by the radial distribution function ( Supplementary Fig. 10 ), showing a sharp peak related to H-bonds between O–H (ribose) and C=O (NDPA) at around 2 Å for both NDPA-AMP and NDPA-ADP, whereas the radial distribution function between the same group of atoms show that these are much further away (>8 Å) in the case of NDPA-ATP. As both right-handed and left-handed helices share that characteristic, the main interactions biasing the energy balance towards right-handed helices in NDPA-ATP are to be found in the periphery of the stacks, at the level of chiral adenosine moieties. However, owing to large constraints where ATP binds to the zinc-dipicolylethylenediamine receptors, slight changes in the conformation of these rigid parts of the assemblies and associated changes in long-range interactions involving the adenosine moieties can produce many local minima with energies within a few kcal per mol per molecule span. Because this conformational space is very difficult to explore exhaustively, we prevent ourselves from comparing the energies of left-handed versus right-handed assemblies. The simulated CD spectra using the right-handed 1-3-2 NDPA-ATP assembly show a bisignated signal with zero crossing at 383 nm, with positive and negative maxima located at 398 and 370 nm, respectively ( Fig. 2b ). The comparison of simulated CD spectra based on average traces of MD snapshots on the (M) -NDPA-AMP and (P) -NDPA-ATP shows oppositely bisignated signals, in fair agreement with the experimental spectra. Dynamic helix reversal The multivalent nature of certain chiral phosphate auxiliaries (ATP or ADP) offers an efficient strategy to modulate the handedness of NDPA stacks through competitive replacement of phosphates, provided that the assembly is dynamic. Addition of 1 equivalent of ATP to a solution of AMP- or ADP-bound helical assembly, (M) -NDPA-AMP or (M) -NDPA-ADP ( c =5 × 10 −5 M in aqueous HEPES (2-[4-(2-hydroxyethyl)piperazin-1-yl]ethanesulfonic acid), 1 equivalent of AMP or ADP), resulted in an inversion of CD signal ( vide infra ), suggesting the formation of (P) -NDPA-ATP stacks, by the competitive replacement of AMP or ADP by ATP, thereby reversal of handedness. We envisaged that the unique differential signalling of Cotton effect via stereomutation in the NDPA helix upon binding to different nucleotides could be explored to probe their conversion from ATP to ADP or AMP and vice versa. However, in order to probe the interconversion kinetics of the bound phosphates, the helical assembly must meet a few requirements. First, the stereomutation process in response to phosphate stimuli should not be the rate-determining step (a rapid, dynamic helix reversal of the stacks is essential) and second, there should not be any chiral amplification so that the absolute CD intensity of the assembly, at any given point of time, directly signals the concentration of bound phosphates. The dynamic nature of the helix reversal in NDPA assemblies was investigated using competitive guest binding. Thus, CD intensity of (M) -NDPA-AMP and (M) -NDPA-ADP stacks upon addition of small amounts of ATP at regular intervals was monitored at 390 nm, as a function of time. Interestingly, both AMP and ADP bound stacks displayed sharp jumps in CD intensity with each successive addition of ATP ( Fig. 3b , red and green traces). For (M) -NDPA-ADP and NDPA-AMP stacks, the signal reversal occurs through multiple stepwise rise of intensity with each addition of ATP. Furthermore, the change from negative to positive bisignated signal is characteristic of stereomutation and indicates the formation of (P) -NDPA-ATP stacks, by the competitive replacement of ADP or AMP with ATP ( Fig. 3c,d ). Such instantaneous changes in Cotton effects provide strong evidence for fast switching of helicity in these dynamic helices. Furthermore, addition of AMP or ADP to (P) -NDPA-ATP did not show any changes in the CD intensity, as the multivalent ATP cannot be competitively replaced by AMP or ADP (blue trace Fig. 3b , Supplementary Figs 1, 11 and 12 ). Moreover, these transformations could also be probed via the changes in their absorption spectra, as the strength of intermolecular interactions varies with different phosphates. Subsequently, ‘Majority Rules’ like experiments performed with mixture of AP, that is, AMP-ATP or ADP-ATP showed almost linear plot of resultant CD intensity against the mole fraction of guests ( Fig. 3e , Supplementary Fig. 13 ), demonstrating the absence of any chiral amplification effects in phosphate-bound NDPA stacks. Thus, the present dynamic chiral assembly is endowed with two unique properties, fast helical response to replacement of binding phosphates and lack of any chiral amplification, enabling the system with an unprecedented ability to probe real-time hydrolysis kinetics of AP. Figure 3: Dynamic helix reversal and chiral amplification. ( a ) Pictorial representation of helicity reversal in NDPA assembly via competitive binding of multivalent AP. ( b – d ) Stepwise dynamic helix reversal experiments performed by sequential addition of ATP to (M) -NDPA-AMP and (M) -NDPA-ADP assemblies (5 × 10 −5 M NDPA in aqueous HEPES (2-[4-(2-hydroxyethyl)piperazin-1-yl]ethanesulfonic acid) with 1 equivalent of respective phosphates). ( b ) Green and red traces show the sharp jumps in CD signal intensity of (M) -NDPA-AMP and (M) -NDPA-ADP, respectively, monitored at 394 nm, upon sequential addition of ATP, represented by the blue arrows. These sharp rises in CD intensity are characteristic of fast helicity reversal and the formation of (P) -NDPA-ATP stacks, which is further evident from the corresponding CD spectral changes shown in c , d . Horizontal nature of these traces suggest that waiting time does not affect the intensity. Blue trace in b shows the CD intensity of (P) -NDPA-ATP upon sequential addition of AMP at time intervals as indicated by the red arrows. The retention of handedness suggests the inability of AMP to replace the pre-bound ATP molecules. ( e ) ‘Majority rules’ like experiment performed using a mixture of ADP and ATP. The linear fit (red line) of the CD intensity rules out any chiral amplification. Full size image Probing enzymatic ATP hydrolysis by stereomutation Next, we probed the dynamic helicity changes of the NDPA stacks, upon in situ hydrolysis of the bound chiral phosphate molecules. As enzymatic cleavage is one of the simplest methods of phosphate hydrolysis inside living cells, Calf Intestinal Alkaline Phosphatase (CIAP) enzyme was chosen, which is known to dissociate all three forms of AP to adenosine and phosphates. Thus, CIAP (0.21 U ml −1 ) was added to (P) -NDPA-ATP helical stacks and CD signal was monitored (390 nm) as a function of time. Interestingly, the CD signal gradually decreases with time, indicating the decrease in ATP concentration on enzymatic hydrolysis with CIAP. Remarkably, the net CD intensity reverses from positive to negative, where the final signal resembles that of ADP- or AMP-bound NDPA assemblies ( Fig. 4b , state-1→state-2). The formation of (M) -NDPA-ADP or (M) -NDPA-AMP stacks is further obvious from the time-dependent CD spectra of (P) -NDPA-ATP assembly with CIAP (0.84 U ml −1 ) monitored at 20 °C, which showed a gradual inversion of positive to negative bisignated signal through an isodichroic point at 368 nm, suggesting complete reversal of helicity ( Fig. 4c ). This inversion of CD signal with time clearly indicates the dynamic reversal of helical handedness of NDPA stacks as a result of conversion of ATP to ADP or AMP through enzymatic hydrolysis. Furthermore, kinetics of this process with varying concentration of enzyme exhibited fast helix reversals with increasing concentration of enzyme ( Fig. 4b ). This unambiguously proves that the rate of helix-reversal directly reflects the progress of enzymatic hydrolysis reaction. From a supramolecular perspective, this enzymatic hydrolysis also provides an unprecedented strategy to modulate the stereomutation kinetics of helical supramolecular polymers. Rate of stereomutation in ( P )-NDPA-ATP could also be controlled by temperature variation, which indicates faster helicity reversal at higher temperatures following a first-order kinetics ( Fig. 4d , Supplementary Fig. 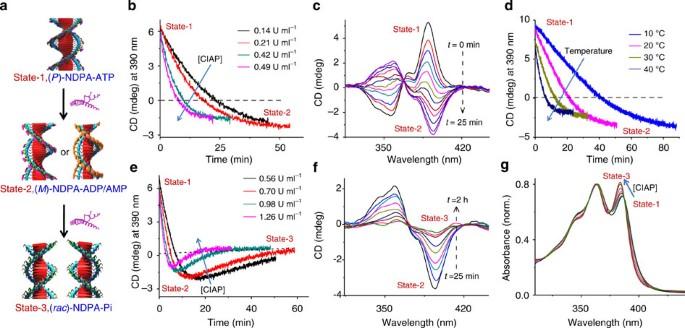Figure 4: Stepwise enzymatic ATP hydrolysis and subsequent dynamic helix reversals. CD kinetic analyses of CIAP triggered stereomutation processes of(P)-NDPA-ATP (c=5 × 10−5M) self-assembly. (a) Schematic illustration of enzymatic action on(P)-NDPA-ATP supramolecular helix (state-1), which first undergoes helix inversion to form(M)-NDPA-ADP and(M)-NDPA-AMP stacks (state-2) followed by racemization to form Pi-stabilized racemic assemblies, (rac)-NDPA-Pi (state-3). (b–d) The spectral changes during the transformation from state-1→state-2 and (e–g) transition from state-2→state-3. (b,e) Time-dependent changes in the CD intensity at 390 nm, with increasing concentration of CIAP at 35 °C. Time-dependent CD spectral changes, upon addition of 0.84 U ml−1of CIAP at 20 °C are shown inc(state-1→state-2) andf(state-2→state-3), whereas ingcorresponding absorption changes (normalized) from state-1→state-3 is presented. (d) Time-dependent changes in the CD intensity (390 nm) of(P)-NDPA-ATP with 0.28 U ml−1of CIAP at varying temperature. Lower CD signal with increasing temperature indis due to weaker ATP binding at elevated temperatures (Supplementary Fig. 15). All experiments were done with one equivalent of AP for better kinetics comparison. Inb, kinetics was not probed for prolonged time to see transition from state-2→state-3. 14 , Supplementary Table 4 ). Figure 4: Stepwise enzymatic ATP hydrolysis and subsequent dynamic helix reversals. CD kinetic analyses of CIAP triggered stereomutation processes of (P) -NDPA-ATP ( c =5 × 10 −5 M) self-assembly. ( a ) Schematic illustration of enzymatic action on (P) -NDPA-ATP supramolecular helix (state-1), which first undergoes helix inversion to form (M) -NDPA-ADP and (M) -NDPA-AMP stacks (state-2) followed by racemization to form Pi-stabilized racemic assemblies, ( rac )-NDPA-Pi (state-3). ( b – d ) The spectral changes during the transformation from state-1→state-2 and ( e – g ) transition from state-2→state-3. ( b , e ) Time-dependent changes in the CD intensity at 390 nm, with increasing concentration of CIAP at 35 °C. Time-dependent CD spectral changes, upon addition of 0.84 U ml −1 of CIAP at 20 °C are shown in c (state-1→state-2) and f (state-2→state-3), whereas in g corresponding absorption changes (normalized) from state-1→state-3 is presented. ( d ) Time-dependent changes in the CD intensity (390 nm) of (P) -NDPA-ATP with 0.28 U ml −1 of CIAP at varying temperature. Lower CD signal with increasing temperature in d is due to weaker ATP binding at elevated temperatures ( Supplementary Fig. 15 ). All experiments were done with one equivalent of AP for better kinetics comparison. In b , kinetics was not probed for prolonged time to see transition from state-2→state-3. Full size image At higher enzyme concentrations (≥0.56 U ml −1 ), (P) -NDPA-ATP showed an interesting phenomenon that apart from the inversion of CD signal in the initial stages, the CD intensity goes to zero at later times and saturates ( Fig. 4e , state-1→state-2→state-3). This clearly suggests two-step process, where ATP is first converted to ADP or AMP leading to reversal of helicity followed by further hydrolysis to adenosine and achiral phosphates thereby loss of chiral information. Moreover, higher CIAP concentration revealed faster kinetics for both these processes, characteristic of enzyme-controlled reaction pathways. The disappearance of CD signal suggests either disassembly of the NDPA stacks in the absence of any bound AP or the formation of racemic stacks stabilized by achiral phosphate Pi, that is, (PO 4 ) 3− produced on hydrolysis. Monitoring the absorption spectra during ATP hydrolysis showed blue shift along with change in ratio of band intensity ( Fig. 4g ). The absorption spectrum after complete stereomutation resemble that of Pi-bound NDPA, thereby ruling out the possibility of NDPA deaggregation ( Supplementary Figs 16 and 17 ). Hence, in the absence of any interactions from CIAP, the final state corresponds to Pi-bound racemic assemblies, that is, ( rac )-NDPA-Pi. Such two-step transitions were not evident at low enzyme concentrations ( Fig. 4b ) as the state-2→state-3 process would take very long time to complete under those conditions. Results thus far have demonstrated that the dynamic helix reversal of the present system can be successfully utilized to probe the enzymatic hydrolysis of ATP and provide useful insights into its stepwise course of action. Moreover, as shown before in Fig. 3b , the CD response to change of phosphates is quiet fast, assuring that the stereomutation closely follow phosphate hydrolysis on the time scale, providing a real-time readout of the enzymatic hydrolysis rates. Insights into enzymatic ATP hydrolysis To gain further insights into various intermediate steps involved in the ATP hydrolysis, similar enzymatic reactions with pure (M) -NDPA-ADP and (M) -NDPA-AMP assemblies were performed. As expected, the time-dependent CD signals monitored at 394 nm gradually goes to zero, suggesting the direct formation of ( rac )-NDPA-Pi assemblies ( Fig. 5 , Supplementary Figs 18 and 19 ). 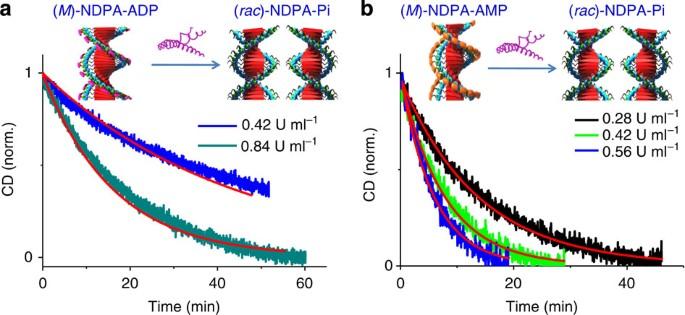Figure 5: Kinetics of ADP and AMP Enzymatic Hydrolysis. Kinetic analyses and comparison of the racemization/helix reversal rates of(M)-NDPA-ADP and(M)-NDPA-AMP stacks. Plot of time-dependent CD intensity monitored at 394 nm showing the racemization process of (a)(M)-NDPA-ADP (c=5 × 10−5M) and (b)(M)-NDPA-AMP (c=5 × 10−5M) to (rac)-NDPA-Pi assemblies, with varying CIAP concentration at 35 °C. The solid lines correspond to their first-order kinetic fits. CD signals were normalized between zero and one for the ease of fitting into kinetic model. First-order kinetic analyses of the decay plots revealed a faster racemization rate for the (M) -NDPA-AMP than that of (M) -NDPA-ADP ( Supplementary Figs 20 and 21 , Supplementary Table 5 ). For example, at 35 °C and with 0.42 U ml −1 of CIAP, the racemization rate constant of (M) -NDPA-AMP ( k amp =0.129 min −1 ), was six times higher than that of (M) -NDPA-ADP ( k adp =0.021 min −1 ), suggesting faster hydrolysis of AMP than ADP. Revisiting the conversion from state-1→state-2 ( Fig. 4e ), as hydrolysis of ADP is much slower than that of AMP, the negative signal at state-2, which is obtained after stereomutation, must be governed mainly by the presence of (M) -NDPA-ADP assemblies. The absorption spectral changes also indicate that state-1→state-2 transformation was governed by ATP→ADP, whereas state-2→state-3 was by ADP→AMP→Pi ( Supplementary Figs 12 and 22 ). The single isodichroic point in the time-dependent CD spectra during stereomutation and their first-order kinetics ( Fig. 4c,d ) further supported that the process is majorly governed by the conversion between two distinct assemblies, (P) -NDPA-ATP and (M) -NDPA-ADP. Thus, dynamic helix reversals in the NDPA supramolecular helical system can be used to probe the mechanistic pathways of enzymatic ATP hydrolysis and possible pathway is via ATP to ADP to AMP before converting to adenosine and phosphates. Moreover, 31 P NMR of ATP in the presence of CIAP also validated the proposed multi-step pathways for enzymatic ATP hydrolysis ( Supplementary Fig. 23 ). Enzymatic action on NDPA-bound phosphate was also monitored by phosphate (Pi) assay using Chen’s method [43] , which corroborated the conclusions drawn from CD kinetic analysis ( Supplementary Fig. 24 ). To further understand the CIAP action, that is, does enzyme selectively hydrolyse the unbound or bound phosphates, CD kinetic measurements of (P) -NDPA-ATP, in the presence of free AMP and ADP molecules, were performed. Absence of an initial lag phase in the resulting kinetic traces rules out any selective action on unbound phosphates ( Supplementary Fig. 25 ). Figure 5: Kinetics of ADP and AMP Enzymatic Hydrolysis. Kinetic analyses and comparison of the racemization/helix reversal rates of (M) -NDPA-ADP and (M) -NDPA-AMP stacks. Plot of time-dependent CD intensity monitored at 394 nm showing the racemization process of ( a ) (M) -NDPA-ADP ( c =5 × 10 −5 M) and ( b ) (M) -NDPA-AMP ( c =5 × 10 −5 M) to ( rac )-NDPA-Pi assemblies, with varying CIAP concentration at 35 °C. The solid lines correspond to their first-order kinetic fits. CD signals were normalized between zero and one for the ease of fitting into kinetic model. Full size image To conclude, we have presented a unique, dynamic, helical assembly that shows AP binding induced supramolecular chirality with tunable handedness. MD simulations suggested different helical supramolecular organizations for NDPA-AMP or NDPA-ADP when compared with NDPA-ATP. With (M) -NDPA-AMP and (M) -NDPA-ADP, the ribose moieties are located very close to the NDI cores, which stabilizes these helices through weak van der Waals and H-bonding interactions. The situation is opposite for NDPA-ATP given the unexpected tendency for ATP to bind Zn atoms in a 1-3-2 motif, resulting in assemblies with ribose moieties pointing away, and no H-bonds with the NDI cores. Furthermore, we show a fast and dynamic switching of helicity through competitive replacement of AMP or ADP by multivalent ATP molecules. This stimuli-responsive helical system with instantaneous reversal of handedness has been utilized for in situ monitoring the kinetics of enzymatic hydrolysis of AP. Detailed kinetic analyses provided insights into mechanistic aspects of this enzymatic hydrolysis process. A clear understanding of the kinetics involved in various processes makes the present system unique for probing phosphates interconversion kinetics. In addition, this system presents an interesting example where the rate of stereomutation can be modulated by an external stimulus such as enzyme. Such a design of dynamic helical assemblies, which responds to biological energy currency, can be envisaged for sensing applications in living cells. Measurements Electronic absorption spectra were recorded on a Perkin Elmer Lambda 900 UV–vis-NIR Spectrometer (Perkin Elmer). Ultraviolet–visible spectra were recorded in 10 mm path length cuvettes. Circular dichroism measurements were performed on a Jasco J-815 spectrometer where the sensitivity, time constant and scan rate were chosen appropriately. Corresponding temperature-dependent measurements were performed with a CDF—426S/15 Peltier-type temperature controller with a temperature range of 263–383 K and adjustable temperature slope. NMR spectra were obtained with a Bruker AVANCE 400 (400 MHz with respect to 1 H nuclei) Fourier transform NMR spectrometer with chemical shifts reported in parts per million. Sample preparation Aqueous HEPES buffer was prepared by making 10 mM solution of HEPES (2-[4-(2-hydroxyethyl)piperazin-1-yl]ethanesulfonic acid) in water. All samples for spectroscopic measurements were prepared by injecting the 5 × 10 −3 M stock solution of NDPA into required volume of aqueous HEPES buffer. Required amount of phosphates were injected into it and the solution was mixed by manual stirring before measurements. Commercially available CIAP was 2.8 U mg −1 and stock solution of CIAP was prepared by dissolving 1 mg of CIAP in 80 μl of aqueous HEPES buffer. Each enzyme kinetic measurements were performed by adding appropriate amount of CIAP stock solution into the phosphate-bound helical stacks at a given temperature and all measurements were initiated immediately. Stepwise dynamic helix reversal measurements in Fig. 3b were performed by injecting aliquots of corresponding phosphates at regular interval to phosphate pre-bound helical stack. (P) -NDPA-ATP term used in the manuscript refers to 5 × 10 −5 M solution of NDPA (in 10 mM aqueous HEPES buffer) with 1 equivalent of ATP. Similarly, ADP-, AMP- and Pi (PO 4 ) 3− -bound helical stacks were denoted as (M) -NDPA-ADP, (M) -NDPA-AMP and ( rac )-NDPA-Pi, respectively. All CIAP-based hydrolysis kinetics of AMP, ADP and ATP were studied with 1 equivalent of respective APs for the ease of comparison. Phosphate’s assay by Chen’s method Chen’s reagent was prepared by adding 1:1:1:2 solution of 10% ascorbic acid (w/v), 2.5% ammonium molybdate (w/v), 6 N H 2 SO 4 and water, respectively. A 5 × 10 −5 M solution of NDPA pre-bound with the appropriate phosphates were treated with suitable amount of CIAP at 35 °C. At regular time interval, 250 μl aliquot of the above solution was added to 1 ml of Chen’s reagent with proper mixing. All such solutions were incubated for 30 min at 35 °C and then absorbance was recorded at 820 nm. This absorbance corresponds to the reduced form of phosphomolybdate complex (formed by Pi released during hydrolysis reaction). Molecular modelling simulations Stacks of NDPA linked to either AMP, ADP or ATP were modelled with the Materials Studio 6.0 modeling package (Accelrys), by MM and MD methods using an in-house adapted version of Dreiding as a force field [44] . To maintain full complexation in NDPA during MD, a bond between the sp 3 nitrogen atom and the zinc atom had to be built. The Dreiding force field was accordingly adapted, increasing the (N_3-Zn) equilibrium distance from 2.022 to 2.585 Å, and replacing the *-Zn-* angle bending term by new angle bending terms, Cl-Zn-Cl, Cl-Zn-N_R, O_3-Zn-O_3, O_3-Zn-N_R and N_R-Zn-N_R, with the same constants as those for *-Zn-*. These adaptations and the validation of the new force field were based on a NDPA structure optimized from density functional theory (DFT) calculations at the B3LYP/6–31G* level, using the LANL2DZ effective core potential and associated basis set to describe the zinc ion. For ATP-based systems, owing to a number of binding possibilities with different orders of binding, that is, 1-2-3 or 1-3-2, isolated trimers were built and optimized, before stacking them into supramolecular assemblies of 33 molecules (11 trimers). For AMP- and ADP-based systems, supramolecular assemblies of 32 molecules were directly built. The initial distance between NDPA planes in the stacks is initially about 3.8 Å and the angle between the molecular axis of neighbouring molecules is set to a value typically between 30° and 60° to avoid steric crowding of the side groups. These assemblies were optimized by MM, and submitted to a 100-ps relaxation Molecular Dynamics with the NDPA cores frozen, to relax most of the steric constraints in the periphery of the assembly, while avoiding disorganizing the stack. Then, a production MD is performed without any constraint during 20 ns. The MM energy minimizations were performed with a conjugate gradient algorithm until a convergence criterion of 0.001 kcal per mol.Å was reached. The long-range interaction cutoff distance was set to 14 Å with a spline width of 3 Å. The charges on the atoms were assigned from the polymer consistent force field (PCFF) [45] , [46] , and tested as previously reported on other types of structures [47] . The MD simulations were performed in the canonical (N,V,T) ensemble. The Nosé thermal bath coupling [48] was used to maintain the temperature at 300 K, with a coupling constant of 0.05. The Verlet velocity algorithm was used to integrate the equations of motion with a 1-fs time step. MM/MD simulations were performed using a distance-dependent dielectric constant as implicit water solvent model. How to cite this article: Kumar, M. et al . A dynamic supramolecular polymer with stimuli-responsive handedness for in situ probing of enzymatic ATP hydrolysis. Nat. Commun. 5:5793 doi: 10.1038/ncomms6793 (2014).